Improving the photovoltage of Cu2O photocathodes with dual buffer layers Cuprous oxide (Cu 2 O) is a promising oxide material for photoelectrochemical water splitting (PEC), and increasing its photovoltage is the key to creating efficient overall PEC water-splitting devices. Previous reports are mostly focused on optimizing the energy band alignment between Cu 2 O and the n-type buffer layer to improve the photovoltage of Cu 2 O photocathodes. However, the band alignment between the n-type buffer layer and the protective layer is often ignored. In this work, Cu 2 O photocathodes with a single buffer layer (Ga 2 O 3 ) and dual buffer layers (Ga 2 O 3 /ZnGeO x ) are fabricated, and their PEC performances are compared. Results show that after inserting the second buffer layer (ZnGeO x ), the onset potential of the Cu 2 O photocathode increases by 0.16 V. Operando electrochemical impedance spectroscopy measurements and analysis of the energy-level diagrams of each layer show that an energy level gradient between Ga 2 O 3 and TiO 2 is created when ZnGeO x is introduced, which eliminates the potential barrier at the interface of Ga 2 O 3 /TiO 2 and improves the photovoltage of the Cu 2 O photocathode. Our work provides an effective approach to improve the photovoltage of photoelectrodes for solar water splitting by introducing dual buffer layers. Solar fuels play a crucial role in the transition from fossil fuel-derived energy to sustainable energy [1] , [2] , [3] . Hydrogen is clean and has a high energy density, these properties make it a key candidate for use as a sustainable fuel [4] , [5] . A transition to sustainable hydrogen fuel will contribute greatly toward the development of a low carbon circular economy and achieving net-zero emissions [6] . Photoelectrochemical (PEC) water splitting can solve the problem of solar energy harvest and storage [7] by converting intermittent solar energy into hydrogen fuel [8] , [9] , which has received great attention in the past decades [10] , [11] . Metal oxides are cost-effective materials for producing photoelectrodes to unlock the potential of photoelectrochemical (PEC) water splitting [12] , [13] . At present, cuprous oxide (Cu 2 O) is one of the best photocathode materials [14] and has attracted great interest due to its inherent p-type character [15] , [16] , natural abundance and low-cost fabrication processes. In addition, its direct bandgap of ~2 eV and appropriate band positions for H 2 evolution make Cu 2 O a primary choice among low-cost photocathode materials [17] . It is difficult to achieve unassisted sunlight-driven water splitting using a single Cu 2 O photocathode [18] , [19] . In general, a self-biased tandem device consisting of the Cu 2 O photocathode and a photoanode or a photovoltaic cell generally needs to be constructed [20] , [21] . For this tandem system, the key to improving the solar to hydrogen (STH) conversion efficiency is to increase the current density at the point where the J-V curves of the photocathode and the photoanode or the photovoltaic cell intersect [22] . Therefore, optimizing the onset potential for the hydrogen evolution reaction (HER) and fill factor of the Cu 2 O photocathode is imperative [20] , [21] . The onset potential is mainly determined by the photovoltage of Cu 2 O and the overpotential of the HER. A larger photovoltage allows the Cu 2 O photocathode to operate at a more positive bias voltage. When Cu 2 O is in direct contact with the electrolyte, a semiconductor-liquid junction (SCLJ) is created. In this situation, the photovoltage is low (<0.6 V) [23] , [24] and photo-corrosion is unavoidable [25] , [26] . Therefore, a buried solid/solid junction was proposed to further increase the photovoltage of the Cu 2 O photocathode and to inhibit photo-corrosion by preventing it from contacting the electrolyte [27] . In early reports, TiO 2 was coupled with Cu 2 O to form a buried junction, but the obtained photovoltage was only 0.46 V [28] , which is mainly due to the limited degree of band-bending of Cu 2 O and the large conduction band offset ( △ E c ) [29] , [30] . Following this, the strategy of adding a dipole layer at the interface between Cu 2 O and TiO 2 was proposed to increase the band-bending of Cu 2 O [31] . However, the improvement in photovoltage was relatively limited. In practice, the photovoltage is determined by the quasi-Fermi levels of the electrons and holes at the interfaces during illumination [29] . Therefore, the n-type semiconductor coupled with Cu 2 O needs to have suitably aligned energy levels [20] , [30] , [32] . After continuous efforts, a variety of n-type buffer layers have been developed, such as Al:ZnO [33] , ZnS [24] , GaN [34] , Ga 2 O 3 [20] , [35] , [36] , and covalent triazine frameworks (CTF-BTh) [37] , which have successfully increased the photovoltage of the Cu 2 O photocathode from 0.5 V to 1 V (vs. RHE). It is also worth noting that Minami et al. focused on the development of new buffer layers (such as ZnMgO, AlGaO and ZnGeO) and the optimization of the p-n junction, which made an important contribution to improving the photovoltage of the Cu 2 O solar cell [38] , [39] , [40] , [41] . In addition, they also emphasized the importance of buffer layer preparation methods [42] . Indeed, for the Cu 2 O photocathode containing a buried junction, the most ideal solution for improving the photovoltage is to construct a homogeneous Cu 2 O p-n junction, which has an approximately equal electron affinity and reduces interfacial lattice mismatches [43] , [44] . However, self-compensation makes it challenging to prepare n-type Cu 2 O with excellent photoelectronic properties [30] . Although numerous attempts have been made, the enhancement of photovoltage in the Cu 2 O photocathode is still insufficient [45] . Moreover, in terms of increasing the photovoltage, the influence of defects and crystal orientation of Cu 2 O cannot be ignored. For example, eliminating interface defects, such as Cu 2+ , has been shown to significantly increase the photovoltage of Cu 2 O-based devices, as it eliminates adverse interfacial defect levels [32] , [46] . Recently, Niu et al. found that when the Cu 2 O with a high index facet group was used in combination with Ga 2 O 3 , it resulted in a larger photovoltage [47] . In brief, previous strategies for increasing the photovoltage of Cu 2 O-based devices are mainly focused on improving the band alignment of the p-n junction interface and reducing the defects in Cu 2 O. In essence, it is mainly about optimizing the band alignment of the interface between Cu 2 O and the n-type buffer layer. For a buried junction, after introducing the n-type buffer layer and the protective layer, it is inevitable that an additional interface is formed between the buffer layer and the protective layer. However, the interfacial effects of n-type layers are often ignored. Recently, Moehl et al. found that in addition to the surface properties of Cu 2 O, the interface of Ga 2 O 3 /TiO 2 also limits the PEC performance of Cu 2 O photocathodes [48] . Therefore, optimizing the band alignment between n-type layers is also important. In this study, by testing the electrochemical impedance spectroscopy under operando conditions, we found that a potential barrier exists at the interface of Ga 2 O 3 /TiO 2 , which decreases the photovoltage and fill factor of the Cu 2 O photocathode. Next, we inserted a second buffer layer (ZnGeO x ) between Ga 2 O 3 and TiO 2 to form an energy level gradient, which eliminates the potential barrier and improves the band alignment. As a result, the photovoltage of the Cu 2 O photocathode was successfully increased from 0.91 to 1.07 V (vs. RHE). Our work provides an effective approach to improve the photovoltage of photoelectrodes for PEC water splitting. Device structure and characterization To prepare the Cu 2 O photocathode, a Cu 2 O thin film was first electrodeposited onto a gold-coated FTO substrate. Next, the conformal Ga 2 O 3 and ZnGeO x buffer layers were deposited on the freshly prepared Cu 2 O film by atomic layer deposition (ALD), followed by the deposition of a TiO 2 protective layer. Finally, the hydrogen evolution catalyst RuO x was deposited by photoelectrochemical deposition (details can be found in the experimental section). The device structure of the Cu 2 O photocathode with dual buffer layers is shown in Fig. 1a . The conformal Ga 2 O 3 layer directly contacts the Cu 2 O film to form a p-n junction. The control photocathode with a single Ga 2 O 3 buffer layer (Cu 2 O/Ga 2 O 3 /TiO 2 ) is prepared in the same way as that of the photocathode with dual buffer layers (Cu 2 O/Ga 2 O 3 /ZnGeO x /TiO 2 ), except that it lacks the ZnGeO x layer. The phase and crystal structure of the obtained photocathodes were characterized by X-ray diffraction (XRD). As shown in Fig. 1b , the XRD patterns indicate that the Cu 2 O is a polycrystalline film with an apparent [111] preferential orientation and it has a cubic structure (PDF #05-0667). The diffraction peaks located at 29.5°, 36.4°, 42.3°, 61.3°, and 73.5° correspond to the (110), (111), (200), (220), and (311) crystal planes, respectively. After the deposition of Ga 2 O 3 , ZnGeO x and TiO 2 layers, no new diffraction peaks were detected, indicating that the Ga 2 O 3 and ZnGeO x buffer layers and the TiO 2 protective layer are amorphous. Fig. 1: Structure, XRD patterns and SEM imaging of the Cu 2 O photocathodes. a A schematic illustration of the structure of the Cu 2 O photocathode with dual buffer layers (Ga 2 O 3 and ZnGeO x ). b XRD patterns of the different films. The diffraction peaks marked with hearts, clubs and diamonds belong to Cu 2 O, Au and FTO, respectively. c Top-view SEM images of the Cu 2 O/Ga 2 O 3 /TiO 2 photocathode. d Top-view SEM images of the Cu 2 O/Ga 2 O 3 /ZnGeO x /TiO 2 photocathode. Full size image In order to visually observe the morphology, thickness and composition of the photocathodes, scanning electron microscopy (SEM), transmission electron microscopy (TEM) and corresponding elemental mapping were carried out. As shown in Fig. 1 c, d , the Cu 2 O/Ga 2 O 3 /TiO 2 photocathode and the Cu 2 O/Ga 2 O 3 /ZnGeO x /TiO 2 photocathode exhibit similar morphology and grain size. Both are thin films composed of assembled cubic particles with a grain size of approximately 300–500 nm. Meanwhile, from the top-view SEM images, the morphology of the films for the Cu 2 O/Ga 2 O 3 /TiO 2 photocathode and the Cu 2 O/Ga 2 O 3 /ZnGeO x /TiO 2 photocathode display similar triangular planes, which implies the [111] preferential orientation of Cu 2 O. This result is consistent with the XRD results. The cross-sectional SEM images (Supplementary Fig. 2 ) clearly show that the thicknesses of the Cu 2 O/Ga 2 O 3 /TiO 2 photocathode and the Cu 2 O/Ga 2 O 3 /ZnGeO x /TiO 2 photocathode are ~904 nm and ~928 nm, respectively. In order to obtain ZnGeO x films with different thicknesses, we deposited the ZnGeO x film using different numbers of super cycles on clean Si substrates. As shown in Supplementary Fig. 4 , the growth rate of ZnGeO x films measured by a step profiler is ~0.55 nm/super-cycle. Therefore, 40 super cycles of ALD result in a ZnGeOx film with a thickness of approximately 22 nm. In addition, as can be observed in the SEM images, after the deposition of the overlayers, the films retain the morphology of Cu 2 O without any aggregation of particles on the surface, indicating that the overlayers cover the Cu 2 O films uniformly and continuously. In order to further examine the heterojunction and multilayer composite structure of the Cu 2 O/Ga 2 O 3 /ZnGeO x /TiO 2 photocathode, TEM and the corresponding elemental mapping were conducted and are depicted in Fig. 2b–k . From the elemental mapping images, Au, Cu, Ga, Zn/Ge, and Ti are detected from bottom to top in the Cu 2 O photocathode, indicating that the device structure is composed of layers. Evidence of the layered structure can also be seen from the line profiles for Ti, Zn, Ge, Ga and Cu elements across the TiO 2 , ZnGeO x , and Ga 2 O 3 /Cu 2 O interfaces (Supplementary Fig. 5 ). The elements in each layer are evenly distributed and in close contact, implying the formation of a close contact buried p-n junction. Furthermore, the uniform distribution of Ge and its position in the same space as Zn indicate that Ge is uniformly doped into ZnO (Fig. 2k ). The elemental mapping images further prove that the overlayer coatings are homogeneous and conformal. We conducted the X-ray photoelectron spectroscopy (XPS) measurements to analyze the chemical composition of ZnGeO x films (Supplementary Fig. 6 ). The atomic ratio of Zn, Ge and O was found to be approximately 21.57:10.64:44.46, which is close to 2:1:4. Therefore, the approximate chemical formula of the ZnGeO x is Zn 2 GeO 4 , and the following ZnGeO x are shorthand for Zn 2 GeO 4 . Fig. 2: SEM and TEM analysis of the Cu 2 O/Ga 2 O 3 /ZnGeO x /TiO 2 photocathode. a Cross-sectional SEM image. b Cross-sectional STEM bright-field image. c Cross-sectional STEM bright-field image of the top of the Cu 2 O/Ga 2 O 3 /ZnGeO x /TiO 2 photocathode. d The STEM high-angle annular dark-field image. e – j Corresponding elemental mapping images of Au, Cu, Ga, Zn, Ge and Ti, respectively. k Combined elemental mapping image of Au, Cu, Ga, Zn, Ge and Ti. Full size image PEC performance and Faradaic efficiency In order to enhance the PEC performance of the Cu 2 O photocathodes, we deposited RuO x as the HER cocatalyst on the surface of the photocathodes using photoelectrochemical deposition. For all the photocathodes, PEC measurements were performed in a phosphate–sulfate buffer electrolyte (pH 5) under simulated AM 1.5 G solar illumination (100 mW cm −2 ) in a standard three-electrode system. Steady-state current-voltage measurements were conducted to evaluate the performance of the Cu 2 O photocathodes. As can be seen in Fig. 3a , the J-V curves tested under chopped illumination show rapidly increased current density, which proves the excellent photo response of all the Cu 2 O photocathodes. Meanwhile, the saturated photocurrent density values for the Cu 2 O/Ga 2 O 3 /TiO 2 and Cu 2 O/Ga 2 O 3 /ZnGeO x /TiO 2 photocathodes are almost the same (5 mA cm −2 ), which is attributed to the same thickness of the Cu 2 O absorber and the same p-n junction interface (Cu 2 O/Ga 2 O 3 ). Compared with the Cu 2 O photocathode comprised of a single buffer layer (Cu 2 O/Ga 2 O 3 /TiO 2 ), the Cu 2 O photocathode with dual buffer layers (Cu 2 O/Ga 2 O 3 /ZnGeO x /TiO 2 ) has a slightly higher fill factor. Fig. 3: Photoelectrochemical measurements. a J-V curves of different Cu 2 O-based photocathodes under simulated AM 1.5 G chopped illumination. b J-V curves of different Cu 2 O-based photocathodes under continuous illumination (AM 1.5 G, 100 mW cm −2 ). c Statistical onset potential of different Cu 2 O-based photocathodes. In this plot, boxes represent the interquartile range or the middle half of the values in each group, and the middle lines in each box represent the medians. The lines coming out from each box extend from the maximum to the minimum values of each set; the whiskers show how big a range there is between those two extremes. When data points go above or below 1.5 times the size of the box, they are outliers and they are dotted outside the whiskers. d Wavelength-dependent IPCE and the integrated current density of the Cu 2 O photocathodes. e The Faradaic efficiency measurement of the Cu 2 O/Ga 2 O 3 /ZnGeO x /TiO 2 photocathode for hydrogen evolution at 0 V RHE under simulated AM 1.5 G irradiation (100 mW cm −2 ). Here, HER stands for hydrogen evolution reaction. RHE stands for reversible hydrogen electrode. f The stability measurement of the Cu 2 O/Ga 2 O 3 /ZnGeO x /TiO 2 photocathode at 0 V RHE under simulated AM 1.5 G irradiation (100 mW cm −2 ). All measurements were performed in pH 5.0 phosphate–sulfate electrolyte. Full size image Here, we define the onset potential as the potential value corresponding to the intercept between the extrapolated tangent lines of the J-V curves measured during illumination (AM 1.5 G, 100 mW cm −2 ) and in the dark (Supplementary Fig. 7 ). In addition, when the bias becomes more negative, the photocurrent density should increase continuously. As shown in Fig. 3b , the onset potential of the Cu 2 O/Ga 2 O 3 /ZnGeO x /TiO 2 photocathode is 1.07 V (RHE), which is positively shifted by 0.16 V (RHE) relative to that of the Cu 2 O/Ga 2 O 3 /TiO 2 photocathode (0.91 V vs. RHE). The statistical data of the onset potential for different batches of Cu 2 O photocathodes (Fig. 3c ) further verifies that inserting the second ZnGeO x buffer layer between the Ga 2 O 3 layer and the TiO 2 layer can increase the photovoltage of the Cu 2 O photocathode. In order to rule out the possibility that the single ZnGeO x buffer layer could improve the onset potential, we also prepared a control photocathode (Cu 2 O/ZnGeO x /TiO 2 ) with the same Cu 2 O thickness and tested its PEC performance. From the results depicted in Fig. 3a–c , the Cu 2 O/ZnGeO x /TiO 2 photocathode shows a lower saturated photocurrent density (~4.7 mA cm −2 ), a later onset potential (0.84 V vs. RHE) and a poor fill factor. After depositing the dual buffer layers, the total thickness of Ga 2 O 3 and ZnGeO x is approximately 40 nm. Since the onset potential is relatively sensitive to the thickness of the buffer layer, we also compared the onset potentials of the Cu 2 O/Ga 2 O 3 -40nm/TiO 2 photocathode and the Cu 2 O/Ga 2 O 3 −20nm/ZnGeO x /TiO 2 photocathode. The results are shown in Supplementary Fig. 8a, b . The onset potential of the Cu 2 O/Ga 2 O 3 −20nm/ZnGeO x /TiO 2 photocathode is still better than that of the Cu 2 O/Ga 2 O 3 -40nm/TiO 2 photocathode (0.95 V vs. RHE), further proving that the dual buffer layers lead to the improvement of the onset potential. When comparing the incident photon-to-current conversion efficiency (IPCE) of Cu 2 O photocathodes consisting of a single buffer layer (Ga 2 O 3 ) and dual buffer layers (Ga 2 O 3 /ZnGeO x ), it can be seen that both show similar trends, as shown in Fig. 3d . In the wavelength region from 350 nm to 480 nm, all the Cu 2 O photocathodes have a high quantum efficiency. However, when the wavelength is longer than 480 nm, the IPCE values drop sharply. Furthermore, compared with the Cu 2 O/Ga 2 O 3 /TiO 2 photocathode, the IPCE of the Cu 2 O/Ga 2 O 3 /ZnGeO x /TiO 2 photocathode is enhanced in the wavelength region from 350 to 480 nm, reaching a maximum of up to 69%. Stability is an important criterion of Cu 2 O photocathodes. Next, we carefully measured the Faradaic efficiency and the stability of the Cu 2 O/Ga 2 O 3 /ZnGeO x /TiO 2 photocathode. To determine the Faradaic efficiency for hydrogen evolution, PEC water-splitting experiments were carried out in a gas-tight H-cell under continuous illumination (AM 1.5 G, 0 V vs. RHE) and the generated hydrogen was measured using an online gas chromatograph. As shown in Fig. 3e , although the values of the Faradaic efficiency fluctuate due to the irregular release of bubbles and small cell headspace, the average Faraday efficiency is close to 100%, indicating that the photogenerated electrons from Cu 2 O photocathode are all used to reduce protons to produce hydrogen. Figure 3f shows the photocurrent density versus time plots under continuous illumination (0 V vs. RHE). The Cu 2 O photocathode with dual buffer layers showed excellent stability over 10 h. The decrease and fluctuation of the photocurrent density in the first 3 h are mainly caused by the attached bubbles on the surface of the Cu 2 O photocathode. 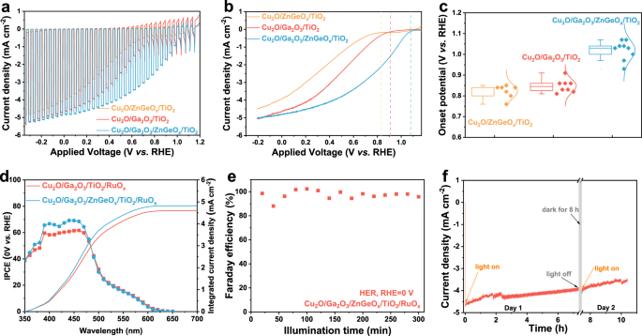Fig. 3: Photoelectrochemical measurements. aJ-Vcurves of different Cu2O-based photocathodes under simulated AM 1.5 G chopped illumination.bJ-Vcurves of different Cu2O-based photocathodes under continuous illumination (AM 1.5 G, 100 mW cm−2).cStatistical onset potential of different Cu2O-based photocathodes. In this plot, boxes represent the interquartile range or the middle half of the values in each group, and the middle lines in each box represent the medians. The lines coming out from each box extend from the maximum to the minimum values of each set; the whiskers show how big a range there is between those two extremes. When data points go above or below 1.5 times the size of the box, they are outliers and they are dotted outside the whiskers.dWavelength-dependent IPCE and the integrated current density of the Cu2O photocathodes.eThe Faradaic efficiency measurement of the Cu2O/Ga2O3/ZnGeOx/TiO2photocathode for hydrogen evolution at 0 VRHEunder simulated AM 1.5 G irradiation (100 mW cm−2). Here, HER stands for hydrogen evolution reaction. RHE stands for reversible hydrogen electrode.fThe stability measurement of the Cu2O/Ga2O3/ZnGeOx/TiO2photocathode at 0 VRHEunder simulated AM 1.5 G irradiation (100 mW cm−2). All measurements were performed in pH 5.0 phosphate–sulfate electrolyte. 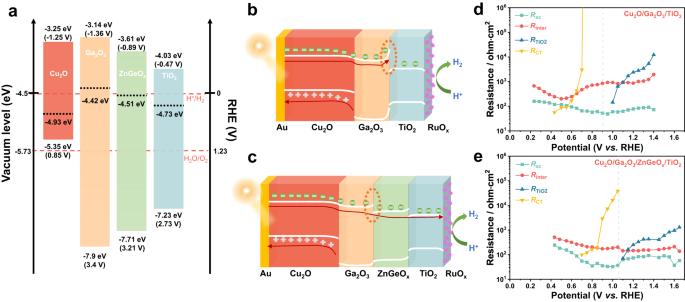Fig. 4: Energy diagrams and extracted resistance. aEnergy diagrams of Cu2O, Ga2O3, ZnGeOx, and TiO2(from left to right) derived from Kelvin probe force microscopy (KPFM), XPS valence-band spectra and the Tauc plots.bSchematic diagram of the photogenerated carrier transport behavior in the Cu2O/Ga2O3/TiO2/RuOxphotocathode under illumination.cSchematic diagram of the photogenerated carrier transport behavior in the Cu2O/Ga2O3/ZnGeOx/TiO2/RuOxphotocathode under illumination.dResistances from the EIS fitting of the Cu2O/Ga2O3/TiO2/RuOxphotocathode under illumination.eResistances from the EIS fitting of the Cu2O/Ga2O3/ZnGeOx/TiO2/RuOxphotocathode under illumination. Deducing the mechanism responsible for the improvement in onset potential After proving that dual buffer layers can improve the HER onset potential, it is important to identify the underlying mechanism. The HER onset potential is determined by the photovoltage and overpotential. Since the same HER catalyst (RuO x ) and the same electrolyte were used to evaluate the PEC performance of all the Cu 2 O photocathodes, the improvement in the onset potential was mainly due to the increased photovoltage rather than the improvement in overpotential. Moreover, the open-circuit potential curves (Supplementary Fig. 10 ) show that the open-circuit potential difference of the Cu 2 O/Ga 2 O 3 /ZnGeO x /TiO 2 /RuO x photocathode (620 mV) is larger than that of the Cu 2 O/Ga 2 O 3 /TiO 2 /RuO x photocathode (450 mV) and the Cu 2 O/ZnGeO x /TiO 2 /RuO x photocathode (390 mV), which further suggests that the Cu 2 O/Ga 2 O 3 /ZnGeO x /TiO 2 /RuO x photocathode possesses an enhanced charge carrier separation efficiency and an increased photovoltage. The photovoltage is related to the defects in Cu 2 O (bulk defects and interfacial defects) and the band alignment optimization of the Cu 2 O photocathode. However, both the Cu 2 O/Ga 2 O 3 /ZnGeO x /TiO 2 and the Cu 2 O/Ga 2 O 3 /TiO 2 photocathodes adopt the same Cu 2 O absorber layer, and the ZnGeO x layer has no direct contact with the Cu 2 O film or RuO x . As a result, the effect of: (1) defects in Cu 2 O and (2) the Cu 2 O/Ga 2 O 3 p-n junction on the optimization of photovoltage are excluded. The only remaining possible cause is that the insertion of the ZnGeO x layer improves the band alignment between Ga 2 O 3 and TiO 2 . We speculate that the ZnGeO x layer provides an energy level gradient between Ga 2 O 3 and TiO 2 , which facilitates the transport of photogenerated electrons and increases the photovoltage of the Cu 2 O photocathode. To confirm our speculation, Fermi levels, valence-band levels and the optical band gaps of each layer in the Cu 2 O/Ga 2 O 3 /ZnGeO x /TiO 2 photocathode were determined using Kelvin probe force microscopy (KPFM), XPS valence-band spectra and Tauc plots (Supplementary Figs. 11 – 13 ). Specifically, Au with a known work function of 5.1 eV was used to calibrate the work function of the KPFM tip for a clean and conductive surface. Since the contact potential difference (CPD) between the sample and the KPFM tip corresponds to their Fermi level ( E F ) difference, the difference in E F between the sample and Au can be obtained by measuring their CPD. Next, the difference between the valence-band maximum ( E VBM ) and E F can be obtained from the XPS valence spectra and thus we can determine the E VBM . The conduction-band minimum of the samples can also be deduced based on their band gaps. Detailed calculation methods are shown in the experimental section. Finally, the energy-level diagrams of Cu 2 O, Ga 2 O 3 , ZnGeO x and TiO 2 are constructed and shown in Fig. 4a . The Fermi level of ZnGeO x is almost identical to that of Ga 2 O 3 . However, its conduction band minimum lies within that of Ga 2 O 3 and TiO 2 . Therefore, the second buffer layer (ZnGeO x ) does provide an energy level gradient between the Ga 2 O 3 and TiO 2 in the Cu 2 O photocathode. Fig. 4: Energy diagrams and extracted resistance. a Energy diagrams of Cu 2 O, Ga 2 O 3 , ZnGeO x , and TiO 2 (from left to right) derived from Kelvin probe force microscopy (KPFM), XPS valence-band spectra and the Tauc plots. b Schematic diagram of the photogenerated carrier transport behavior in the Cu 2 O/Ga 2 O 3 /TiO 2 /RuO x photocathode under illumination. c Schematic diagram of the photogenerated carrier transport behavior in the Cu 2 O/Ga 2 O 3 /ZnGeO x /TiO 2 /RuO x photocathode under illumination. d Resistances from the EIS fitting of the Cu 2 O/Ga 2 O 3 /TiO 2 /RuO x photocathode under illumination. e Resistances from the EIS fitting of the Cu 2 O/Ga 2 O 3 /ZnGeO x /TiO 2 /RuO x photocathode under illumination. Full size image In order to shed light on how the energy level gradients optimize the band alignment and improve the photovoltage, a powerful non-destructive characterization method is necessary to reveal the underlying transport behavior of the photogenerated electrons through the interface of each layer in the photocathode under operando condition. Recently, Moehl et al. established a resistance-based method using electrochemical impedance spectroscopy (EIS) to identify relevant charge carrier transfer processes under operation [44] . Under illumination, the minority charge carriers dominate the light-induced processes. They investigated the underlying potential-dependent processes during water splitting for the Cu 2 O/Ga 2 O 3 /TiO 2 photocathode and assigned the resistance observed in the EIS spectra under illumination to the relevant charge carrier transfer process, denoted as R CT , R SC , R TiO2 and R inter . Moreover, Moehl et al. concluded that the main limitations of the onset potential for the Cu 2 O/Ga 2 O 3 /TiO 2 photocathode are the adverse barriers present at the Ga 2 O 3 /TiO 2 and TiO 2 /RuO x interface [44] . In order to reveal the underlying transport behavior of the photogenerated electrons through the interface of each layer in the Cu 2 O photocathode, we compared the electrochemical impedance spectra of Cu 2 O/Ga 2 O 3 /TiO 2 and Cu 2 O/Ga 2 O 3 /ZnGeO x /TiO 2 photocathodes, the measurements were conducted under illumination (~120 W m −2 ). The Nyquist plots of both Cu 2 O photocathodes are displayed in Supplementary Fig. 15b–g . The corresponding equivalent circuit model used to fit the Cu 2 O devices is shown in Supplementary Fig. 15a . The resistances of R CT , R SC , R TiO2 and R inter from the EIS fitting procedure were extracted (Fig. 4d, e ). All resistances are present during water splitting. In detail, R CT , the low-frequency resistance, is related to the hydrogen-generating charge transfer over the hydrogen-evolving catalyst (HEC) into the electrolyte solution, implying that Ru(IV) is reduced to Ru(III). R CT is related to the current flow for the reduction step of RuO x . When the bias is more negative than the onset potential for HER, more photogenerated charge carriers reach the electrolyte through RuO x . RuO x will be reduced faster, and the R CT will decrease dramatically. R SC is related to the recombination process of the photogenerated charge carriers. It represents the recombination resistance of the photogenerated electron-hole pairs. Before the bias reaches the onset potential for HER, the electrons flow inside the Cu 2 O photocathode is negligible. Therefore, the R SC is normally constant. However, once the recombination of photogenerated carriers is suppressed, such as when the bias exceeds the onset potential, R SC will increase. R TiO2 is related to a resistive limitation at the TiO 2 /RuO x interface. This resistance is caused by the unfavorable band bending for the contact between TiO 2 and RuO x [44] . Finally, R inter is related to the interfacial defects of Cu 2 O and the interfacial barrier of Ga 2 O 3 /TiO 2 caused by the upward band bending of the conduction band of Ga 2 O 3 (Fig. 4b ). As shown in Fig. 4d, e , the R TiO2 values for Cu 2 O/Ga 2 O 3 /TiO 2 and Cu 2 O/Ga 2 O 3 /ZnGeO x /TiO 2 photocathodes both show an exponential trend in reduction in two segments, indicating the increasing current flow for the reduction of the RuO x catalysts. Before H 2 evolution proceeds, their R SC is almost constant, implying that the flow of electrons inside the Cu 2 O photocathode is negligible. When the reverse bias exceeds the HER onset potential, both of their R SC values increase gradually, which is due to the suppressed recombination of the photogenerated carriers. Furthermore, for the Cu 2 O/Ga 2 O 3 /ZnGeO x /TiO 2 photocathode, the increasing slope of its R SC is larger than that of the Cu 2 O/Ga 2 O 3 /TiO 2 photocathode, indicating that the Cu 2 O/Ga 2 O 3 /ZnGeO x /TiO 2 photocathode has a better fill factor. This is consistent with the results of the measured J-V curves (Fig. 3a, b ). As for the R CT of the Cu 2 O photocathodes with a single buffer layer (Ga 2 O 3 ) and dual buffer layers (Ga 2 O 3 /ZnGeO x ), it shows a steep downward trend, indicating that Ru (VI) is rapidly reduced to Ru(III). The trends observed here for the changes in R CT , R SC , and R TiO2 are consistent with the results presented by Moehl et al. [44] . However, for Cu 2 O/Ga 2 O 3 /TiO 2 and Cu 2 O/Ga 2 O 3 /ZnGeO x /TiO 2 photocathodes, their R inter values show different trends. Both of their R inter values are almost constant before H 2 evolution begins, and the R inter of the Cu 2 O/Ga 2 O 3 /ZnGeO x /TiO 2 photocathode is smaller than that of the Cu 2 O/Ga 2 O 3 /TiO 2 photocathode. After the reverse bias exceeds the HER onset potential, the R inter of the Cu 2 O/Ga 2 O 3 /TiO 2 photocathode decreases initially and then increases gradually. However, the R inter of the Cu 2 O/Ga 2 O 3 /ZnGeO x /TiO 2 photocathode shows a gradually increasing trend without decreasing. According to the analysis results of Moehl et al., the decrease in R inter after passing the HER onset potential is caused by the interfacial barrier of Ga 2 O 3 /TiO 2 [44] . However, when the reverse bias is increased further, R inter will increase again. This process represents the reduced recombination of photogenerated charge carriers. The increase of R inter is caused by the decreasing interfacial barrier of Ga 2 O 3 /TiO 2 , since the increasing reverse bias elevates the conduction band of Ga 2 O 3 and inhibits the upward band bending of Ga 2 O 3 . As for the R inter trend for the Cu 2 O/Ga 2 O 3 /ZnGeO x /TiO 2 photocathode, the decreasing trend disappears. Therefore, it is reasonable to consider that the interfacial barrier in Ga 2 O 3 /TiO 2 is eliminated. As shown in Fig. 4a , since the Fermi levels of Ga 2 O 3 and ZnGeO x are similar, the upward band bending of Ga 2 O 3 is suppressed (Fig. 4c ). As the conduction band level of ZnGeO x lies between that of Ga 2 O 3 and TiO 2 , the insertion of ZnGeO x provides an energy level gradient (Fig. 4c ), improving the band alignment of the Cu 2 O photocathode. As a result, the photogenerated electrons can smoothly transport from Cu 2 O to the RuO x catalysts without any barriers, reducing the interfacial energy loss. Finally, the influence on the J-V curves is shown by the positive shift of the onset potential and the increased fill factor. In summary, here, we demonstrate that inserting a second buffer layer (ZnGeO x ) between the Ga 2 O 3 layer and the TiO 2 layer can improve the onset potential of the Cu 2 O photocathode by 0.16 V. By combining the energy-level diagrams of each layer in the Cu 2 O photocathode with the results obtained from operando electrochemical impedance spectroscopy measurements, we found that the insertion of ZnGeO x introduces an energy level gradient and eliminates the interfacial barrier of Ga 2 O 3 /TiO 2 . As a result, it improves the band alignment and increases the photovoltage of the Cu 2 O photocathode. Our work provides an effective approach to increase the photovoltage of photoelectrodes with buried junctions. In this work, we have shown that the construction of dual buffer layers in the Cu 2 O photocathode can increase the photovoltage to 1.07 V. However, given that the bandgap of Cu 2 O is 2 eV, the theoretical maximum photovoltage of the Cu 2 O photocathode can reach 1.6 V [49] , which leaves a lot of space for further improvement of its photovoltage. In addition to optimizing the band alignment between the n-type buffer layer and the protective layer, it is important to optimize the band alignment of the p-n junction interface. For transparent n-type layers coupled with Cu 2 O, there should be a larger Fermi level difference and a smaller conduction band offset relative to Cu 2 O. In addition, n-typer layers should have excellent electrical conductivity. Up until now, Ga 2 O 3 is still one of the best n-type buffer layers for the Cu 2 O photocathode. However, insulator-like Ga 2 O 3 has a larger resistance, which is not conductive to the transport of charge carriers. Increasing the carrier densities and conductivity of Ga 2 O 3 by heteroatom doping may be an effective solution [32] . In addition, the influence of interfacial defects or surface states on the photovoltage of the Cu 2 O photocathode cannot be ignored. These defects, such as Cu 0 or Cu 2+ , can narrow the splitting of the quasi-Fermi level and trigger the recombination of hole-electron pairs by restricting the Fermi level of Cu 2 O, which eventually decreases the photovoltage [29] , [50] . However, the current understanding of defect generation and the specific mechanism affecting the photovoltage is unclear and further investigation is required. The preparation of high-quality single-crystal Cu 2 O is also worth further development and exploration. Finally, the effect of different crystal groups on the photovoltage of Cu 2 O photocathodes is also a very interesting and important research point. Chemicals All the chemicals and reagents were used as purchased without further purification. Chemicals and reagents used in this work are as follows: copper (II) sulfate (≥99.95%, Sigma-Aldrich), DL-Lactic acid (90%, TCI), potassium phosphate dibasic anhydrous (99.99%, Aladdin), potassium hydroxide (99.999%, Aladdin), bis(μ-dimethylamino)tetrakis(dimethylamino)digallium (98%, Strem Chemicals), tetrakis-dimethylamino titanium (99%, Strem Chemicals), diethyl zinc (99.99%, Dongguan NanoFrontier Microelectronic Equipment Co. Ltd), tetramethoxygermane (98%, Alfa Aesar), sodium sulfate anhydrous (99%, Aladdin), potassium dihydrogen phosphate (99.5%, Aladdin), TritonX-100 ( n ≈ 10, Aladdin). Ultrapure water (18.2 MΩ ⋅ cm, Purelab Ultra, ELGA) was used for the preparation of aqueous solutions. Electrodeposition of cuprous oxide (Cu 2 O) All Cu 2 O photocathodes were prepared using FTO coated with a 160 nm Au film as the substrates. In order to enhance the adhesion between the Au film and FTO, a 20 nm Cr film was inserted between them. The Au film and the Cr film were prepared by DC magnetron sputtering. The electroplating solution was a basic solution of lactate-stabilized copper sulfate prepared by dissolving 4 g CuSO 4 , 33.75 g lactic acid and 10.885 g K 2 HPO 4 in 125 mL H 2 O. A 2 M KOH solution was then used to adjust the solution pH to 12. The electrodeposition of Cu 2 O was performed using galvanostatic mode with a current density of −0.1 mA cm −2 in a two-electrode configuration. The electrodeposition time of all Cu 2 O films was 100 min, which resulted in a Cu 2 O film with a thickness of approximately 860 nm. A large piece of frosted glass coated with a thicker Au film was used as the counter electrode. During deposition, the electrolyte was maintained at 30 °C using a hot plate fitted with an in-situ temperature probe. Immediately after the electrodeposition, the surface of the Cu 2 O film was washed with plenty of water and dried with N 2 . Atomic layer deposition of overlayers For all the Cu 2 O photocathodes, all freshly prepared Cu 2 O films were immediately transferred to the atomic layer deposition chamber for subsequent film deposition after being dried with N 2 . A 3 × 7 cm Cu 2 O film substrate was cut into two pieces and put into the same deposition chamber. The ALD-Ga 2 O 3 film was then deposited onto the two Cu 2 O film samples. One sample was then removed and an ALD-ZnGeO x film was deposited on the other sample. Finally, the ALD-TiO 2 protective layer was deposited on the two samples in the same batch to obtain the Cu 2 O/Ga 2 O 3 /TiO 2 device and the Cu 2 O/Ga 2 O 3 /ZnGeO x /TiO 2 device, respectively. As for the preparation of the Cu 2 O/ZnGeO x /TiO 2 device, the ALD-ZnGeO x film and ALD-TiO 2 film were directly deposited on the freshly prepared Cu 2 O film in turn. A portion of the exposed gold substrate was masked with Kapton tape prior to the deposition of the overlayers. The ALD-Ga 2 O 3 film was deposited by running 200 periodic cycles consisting of 1 cycle of bis(μ-dimethylamino)tetrakis(dimethylamino)digallium and water, at 150 °C, which gives a film of approximately 20 nm in thickness. In order to ensure that there was a sufficient amount of Ga in the deposition cavity, the Ga source cylinder was heated at 124 °C. During deposition, the Ga precursor ALD valve was opened for 0.25 s, followed by a 20 s N 2 purge. Germanium-doped zinc oxide (ZnGeO x ) was deposited by running 40 super cycles consisting of 1 cycle of tetramethoxygermane and water after 3 cycles of diethyl zinc and water, at 120 °C, which gives a film of approximately 20 nm in thickness. The Ge precursor ALD valve was opened for 0.18 s, followed by a 15 s N 2 purge. Next, a 0.1 s pulse of H 2 O was used, followed by a 20 s N 2 purge. The Zn precursor ALD valve was opened for 0.07 s, followed by a 15 s N 2 purge. Then a 0.1 s pulse of H 2 O was used, followed by a 20 s N 2 purge. Titanium dioxide (TiO 2 ) was deposited at 150 °C using tetrakis-dimethylamino titanium (TDMAT) and H 2 O as the Ti and O precursors, respectively. The growth rate of the ALD-TiO 2 film was 0.056 nm/cycle. To ensure that the vapor pressure was sufficient, TDMAT was heated to 80 °C. The precursor temperatures of Ge, Zn, and O were kept at room temperature. The ALD process was operated in a thermal ALD system (NCE-200R). For scanning voltammetry testing and the measurement of open-circuit potential, the thickness of the TiO 2 protective layer was 20 nm, while for stability testing and the Faraday efficiency measurements, the thickness of the TiO 2 protective layer was 120 nm. RuO x catalyst photoelectrodeposition Galvanostatic photoelectrodeposition was used to deposit the RuO x catalyst onto the Cu 2 O samples. Typically, RuO x was deposited at a current density of −30 μA cm −2 for 6 min under simulated one sun illumination in a standard three-electrode configuration. The electroplating solution was prepared by dissolving 2.6 mg KRuO 4 in 10 mL H 2 O. Material characterization XRD measurements were performed on a Rigaku X-ray diffractometer using Cu Kα radiation, a scanning range of 2θ = 20–80° and a scan rate of 10° min −1 . 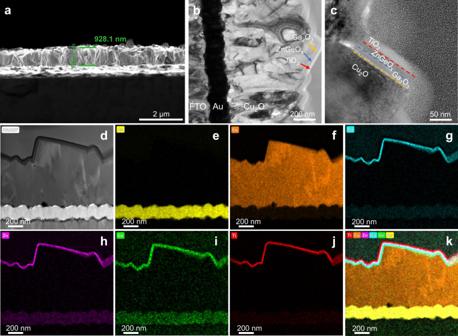The morphology of the films was characterized using a high-resolution scanning electron microscope (Apreo S LoVac). For TEM imaging, the cross-sectional lamellae of the Cu 2 O photocathode samples were prepared using the focused ion beam technique (Helios NanoLab 460HP). Fig. 2: SEM and TEM analysis of the Cu2O/Ga2O3/ZnGeOx/TiO2photocathode. aCross-sectional SEM image.bCross-sectional STEM bright-field image.cCross-sectional STEM bright-field image of the top of the Cu2O/Ga2O3/ZnGeOx/TiO2photocathode.dThe STEM high-angle annular dark-field image.e–jCorresponding elemental mapping images of Au, Cu, Ga, Zn, Ge and Ti, respectively.kCombined elemental mapping image of Au, Cu, Ga, Zn, Ge and Ti. Pt deposition was used to protect the surface. TEM characterization was performed on a TEM (FEI-Talos F200X) operating at 200 kV. Both TEM and STEM modes were used. EDS mapping was acquired by using quadrant EDS detectors in STEM mode. The composition of the ALD-ZnGeOx film was analyzed by X-ray photoelectron spectroscopy (Thermo Fisher Scientific ESCALAB 250Xi). Optical absorption spectra were collected at room temperature with a UV-vis spectrophotometer (UV-2600, Shimadzu). The growth rate of the ALD-ZnGeO x film was tested using a step profiler (Kosaka ET200). Measurements of the XPS valence-band spectra were conducted using a photoelectron spectrometer (Thermo Fisher Scientific ESCALAB 250Xi) featuring monochromatic Al Kα radiation (hν = 1486.68 eV) under a pressure of 1 × 10 −9 mbar. The Fermi level edge of the Au reference film was used to calibrate the binding energy scale. The contact potential difference (CPD) and KPFM images were obtained in an ambient atmosphere using a Bruker Dimension Icon instrument. The CPD between the sample films and the KPFM tip (conductive CoCr-coated Sb-doped Si) can be determined using the following equations [51] , [52] , [53] : 
    -e×V_CPD=W_Tip-W_Film
 (1) 
    E_fFilm=-W_Film
 (2) Where W Tip and W Film are the work functions of the KPFM tip and the as-obtained film, respectively, and E fFilm is the Fermi level of the as-obtained film. In order to determine the Fermi level of the sample films, Au with a known work function of 5.1 eV was used to calibrate the work function of the KPFM tip for a clean and conductive surface. The valence-band maximum ( E VBM ) can be determined using the following equation: 
    E_VBM=E_fFilm-E_edge
 (3) Where E edge is the valence-band edge. E edge can be obtained via extrapolation to the linear part of the binding-energy edge in the XPS valence-band spectra. It represents the difference between E VBM and E fFilm , for each material. Photoelectrochemical analysis Current-voltage measurements were conducted in homemade PEEK cells using a three-electrode configuration, where a Cu 2 O photocathode was the working electrode, Pt plate is the counter electrode and Ag/AgCl/sat. KCl was the reference electrode. A scan rate of 10 mV s −1 in the cathodic direction was used to acquire the data. The electrolyte solution was a pH 5 buffer solution containing 0.5 M Na 2 SO 4 and 0.1 M sodium phosphate. The photoelectrochemical performance of the photocathodes was studied using a CHI-760E electrochemical workstation. Specifically, the photo response of the photocathodes was measured under simulated AM 1.5 G illumination (100 mW cm −2 ) generated from a Xe-lamp (MC-X301B) equipped with an AM 1.5 G filter. The light intensity was controlled by light path distance which is determined by measuring the short-circuit current of a calibrated silicon diode with a KG 3 filter. All potentials have been referenced to the RHE using the following equations: 
    V_RHE=V_Ag/AgCl+0.197 V+0.059 V×pH
 (4) IPCE was measured in a home-built system equipped with a Xe-lamp and a monochromator. Measurements were conducted using a three-electrode configuration at 0 V versus the reversible hydrogen electrode (RHE). Comparison with a calibrated Si photodiode allowed the calculation of the IPCE. Stability and Faradaic efficiency measurement For the stability tests, the Cu 2 O photocathode containing a 120 nm TiO 2 film was inserted in a quartz cell filled with electrolyte, and the change in behavior of the photocurrent density over time was monitored under a constant bias voltage of 0 V (vs. RHE). The measurement was conducted under rapid stirring in a standard three-electrode configuration. The light intensity was calibrated to 100 mW cm −2 . The electrolyte solution was a pH 5 buffer solution, containing 0.5 M Na 2 SO 4 and 0.1 M sodium phosphate. The Faradaic efficiency of the photocathode was measured in a gas-tight photoelectrochemical H-cell under a constant bias voltage of 0 V (vs. RHE), equipped with an anion exchange membrane (Selemion AMVN, AGC Inc.) separating both compartments and with a quartz window (2 cm in diameter). An Ag/AgCl (KCl sat.) reference electrode was employed and a platinum mesh was used as the counter electrode. Ar gas was bubbled through the catholyte at a flow rate of 15 mL min −1 during the measurement. The resulting gas products were passed through the sample loop of a gas chromatograph equipped with a thermal conductivity detector (TCD) and analysis was carried out in 20-min intervals. The light intensity was calibrated to 100 mW cm −2 . The electrolyte solution was a pH 5 buffer solution, containing 0.5 M Na 2 SO 4 and 0.1 M sodium phosphate. The measured amount of hydrogen produced, in moles, was compared to the observed photocurrent density, which provided the Faradaic efficiency. Electrochemical impedance measurements The electrochemical impedance spectroscopy (EIS) measurements were carried out following a previously reported method [48] . In brief, EIS measurements were carried out under illumination (~120 W m −2 ) using a three-electrode configuration in pH 5.0 phosphate–sulfate electrolyte. In order to minimize the size of bubbles formed, 1 mM TritonX was dissolved in the electrolyte. Full impedance spectra were measured using an Autolab M204 at frequencies from 1 MHz to 0.2 Hz. The range of the bias potential was 1.65–0.2 V (vs. RHE). The bias potential steps were 50 mV and the equilibration time at each bias potential step was normally 30 s. The EIS spectra were fitted with Zview. For details about the model used for the fitting procedure, please see below (Supplementary Fig. 15a ). Before each EIS measurement, the device was preconditioned at the starting potential for 180 s to achieve the steady state of the RuO x /electrolyte solution interface. Based on the number of processes observed in the Nyquist plot, a corresponding number of simple resistors and capacitors are used to fit the EIS spectra. Resistors and capacitors corresponding to the same process are connected in parallel, while elements of different processes are connected in series (Supplementary Fig. 15a ). To account for the non-ideality of the capacitors constant phase elements, CPEs, have been used (with the exponent accounting for the ideality of the CPE not going below 0.8). This fitting method could result in a less accurate overview of the photophysical processes. However, the determined resistances and their dependence on the applied potential still enable us to draw valuable conclusions on the operation of the system and the assigning of the resistances to certain photophysical or electrochemical processes. Generally, we can assume that photogenerated charge carriers are subjected to a recombination process inside the space charge region of the photoabsorber. This process normally takes place in the μs range for sufficiently efficient devices and is therefore situated in the HF region of the EIS measurements (MHz down to KHz). 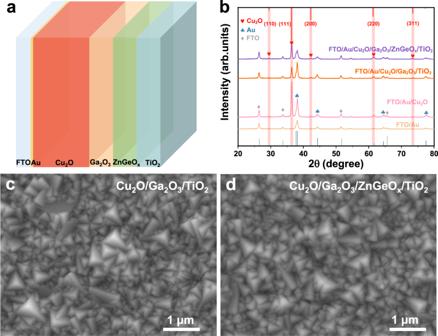The recombination resistance associated with this process will increase when the recombination current is suppressed. Therefore, before the bias reaches the HER onset potential or the recombination is suppressed by strong band bending, the recombination resistance associated with this process is normally constant. As for the slow process associated with the electron charge transfer into the electrolyte, the corresponding resistance in the EIS measurements appears in the mHz to Hz range [48] . Fig. 1: Structure, XRD patterns and SEM imaging of the Cu2O photocathodes. aA schematic illustration of the structure of the Cu2O photocathode with dual buffer layers (Ga2O3and ZnGeOx).bXRD patterns of the different films. The diffraction peaks marked with hearts, clubs and diamonds belong to Cu2O, Au and FTO, respectively.cTop-view SEM images of the Cu2O/Ga2O3/TiO2photocathode.dTop-view SEM images of the Cu2O/Ga2O3/ZnGeOx/TiO2photocathode. The characteristic frequency of each resistance element is displayed in Supplementary Table 1 .